Analysis of deletion breakpoints from 1,092 humans reveals details of mutation mechanisms Investigating genomic structural variants at basepair resolution is crucial for understanding their formation mechanisms. We identify and analyse 8,943 deletion breakpoints in 1,092 samples from the 1000 Genomes Project. We find breakpoints have more nearby SNPs and indels than the genomic average, likely a consequence of relaxed selection. By investigating the correlation of breakpoints with DNA methylation, Hi–C interactions, and histone marks and the substitution patterns of nucleotides near them, we find that breakpoints with the signature of non-allelic homologous recombination (NAHR) are associated with open chromatin. We hypothesize that some NAHR deletions occur without DNA replication and cell division, in embryonic and germline cells. In contrast, breakpoints associated with non-homologous (NH) mechanisms often have sequence microinsertions, templated from later replicating genomic sites, spaced at two characteristic distances from the breakpoint. These microinsertions are consistent with template-switching events and suggest a particular spatiotemporal configuration for DNA during the events. Genome structural variations (SVs) involving hundreds and thousands of bases are common during evolution and are widespread in the human genome [1] , [2] . The larger fraction of the human genome affected by SVs than single-nucleotide polymorphisms (SNPs) [3] implies that they may have greater, or at least similar, consequences for phenotypic variation and evolution than SNPs [1] , [2] . Not surprisingly, SVs can cause and have been associated with numerous diseases [4] , [5] , [6] , [7] , [8] , [9] , [10] . SV occurrence and existence is a complex phenomenon that is not completely understood. SVs, similar to other genomic variants, are genetic imprints of mutational processes in cells. The sequence content of SVs can carry important information about their origin; however, bases around their breakpoints hold the most crucial details of SV genesis. Long homologies around breakpoints suggest SV formation by non-allelic homologous recombination (NAHR); short homologies, with high mobile element content within SV regions, suggest that they originated through transposable element insertions (TEI); while little or no homology (NH) at breakpoints indicates that an SV originated as a result of a non-homologous end-joining (NHEJ) event or by a template-switching mechanism during replication [11] . The latter mechanisms include fork stalling and template switching [12] and microhomology-mediated break-induced replication [13] . Mistakes in breakpoint resolution of just several bases can lead to misclassification of mutational signatures and compromise downstream analysis. Thus, studying SVs at breakpoint resolution is fundamental to understand the mutational mechanisms generating them. A few systematic genome-wide studies of SV breakpoints have been carried out to date [14] , [15] , [16] , [17] . In particular, studies by Lam et al. [14] , Conrad et al. [16] and Kidd et al. [15] , analysed 1,961, 324 and 1,054 SV breakpoints in 14, 3 and 17 individuals, respectively. The majority of SVs analysed in those studies were larger than 1 kbps. Analysis of genomes from 180 individuals in the pilot phase of the 1000 Genomes Project [17] revealed that there are at least an order of magnitude more SVs present in the human population, a significant fraction, if not most, of which are smaller than 1 kbps. The challenge of precise breakpoint identification from inexpensive short-read sequencing was also realized [18] . Along with advances in breakpoint ascertainment, recent multiple studies aimed at deciphering genome function have been conducted that have generated a wealth of functional genomic data. For example, the ENCODE project [19] and The NIH Roadmap Epigenomics Mapping Consortium [20] released data on chromatin marks, methylation, DNase-hypersensitive sites and transcription binding sites in multiple cell lineages and tissues. These data allow the study of SV breakpoints in the context of genome functional and epigenetic contents. Here we describe the discovery and analysis of a large set of 8,943 high confidence deletion breakpoints from 1,092 individuals sequenced in phase 1 of the 1000 Genomes Project [21] . We put special emphasis on the derivation of our set of high-precision breakpoints and provide this data set as a valuable resource for others. Our subsequent downstream analysis, including correlating breakpoints with functional genomic data, reveals important details of their mechanisms of formation and the genomic characteristics associated with them. In particular, we hypothesize that some NAHR deletions occur without DNA replication and suggest that DNA should be in a particular spatial and temporal configuration to generate SVs during a template-switching event. Deriving the confident set of breakpoints We performed comprehensive discovery of deletions [21] , targeted breakpoint assembly [22] and breakpoint mapping with two pipelines [22] , [23] to arrive at a candidate set of breakpoints ( Fig. 1a ). To derive high-quality data set, we needed to address two types of errors: false deletion calls and incorrect breakpoint assembly. Consequently, we developed a dedicated filter that utilized unmapped reads and an empirical null model ( Fig. 1b ). Briefly, the model used inner sequences adjacent to deletion breakpoints to construct junctions simulating random sequences, that is, null sequence junctions. Note that this model imitates biologically relevant sequence homologies around breakpoints. We realigned unmapped reads to real and null junctions and optimized the criteria for considering whether a read supports a junction by interrogating alignments to null junctions, as such alignments reflect random noise (see Methods). 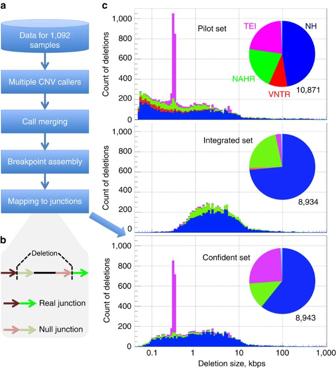Figure 1: Deriving confident set of breakpoints. (a) Conceptual steps for the derivation. Breakpoints from local target assembly are filtered by mapping reads to putative junctions. (b) Null model for breakpoint filtering. (c) Comparison of different breakpoint sets. The pilot set17was included in the derivation as one of the call sets. Integrated set21was biased towards large nonrepetitive deletions for the purpose of reliable genotyping, resulting in the strong under-representation of mobile element insertions. The overlap between confident set and pilot/integrated sets was roughly 50% (Supplementary Fig. 3). Figure 1: Deriving confident set of breakpoints. ( a ) Conceptual steps for the derivation. Breakpoints from local target assembly are filtered by mapping reads to putative junctions. ( b ) Null model for breakpoint filtering. ( c ) Comparison of different breakpoint sets. The pilot set [17] was included in the derivation as one of the call sets. Integrated set [21] was biased towards large nonrepetitive deletions for the purpose of reliable genotyping, resulting in the strong under-representation of mobile element insertions. The overlap between confident set and pilot/integrated sets was roughly 50% ( Supplementary Fig. 3 ). Full size image For validation we performed PCR amplification across breakpoints and tested for differences in intensity values for SNP probes across individuals with and without deletions—the Intensity Rank Sum (IRS) test [17] (see Methods). The final set consisted of 8,943 deletion breakpoints with consistent false discovery rate (FDR) estimates from PCR (6.8%) and IRS (6.4%) validations for deletion existence, and 13.7% for deletion presence with precise breakpoints from PCR. Precision was confounded by repeats around breakpoints. Typically, we observed a shift between breakpoint coordinates from assembly and validation; however, in one case we observed that assembly collapsed repeats ( Supplementary Fig. 1 ). Using a read depth approach, we genotyped 4,384 variants from the set as deletions in two trios sequenced to high coverage by long reads. With these data as supporting evidence we confirmed 3,034 breakpoint sequences (34% of the entire set) and, after minimizing confounding factors, calculated yet another FDR estimate of 18% for deletion presence with precise breakpoints ( Supplementary Data 1 and Methods ). As expected, we find exponentially more of the less frequent deletions, with roughly 54% genotyped in less than 2% of studied individuals ( Supplementary Fig. 2 ). Using OMNI genotyping arrays we estimated that our breakpoint genotyping, while being very precise, misses roughly 60% of samples; the results of shallow 4–8X sequencing limiting coverage of breakpoints to an average of two to four reads. In addition, due to stringent criteria for breakpoint support, breakpoints of rare deletions are less likely to be confirmed by read mapping. As a consequence, the frequency spectrum of deletions in the set was shifted towards more common events as compared with the SNP set discovered from the same data ( Supplementary Fig. 2 ). Overall, our breakpoints are of higher quality than those derived in the pilot phase of the 1000 Genomes Project [17] ( Supplementary Fig. 3 ) and are more representative in their length distribution than those used recently in the following phase [21] ( Fig. 1c ), as the latter set was limited to large nonrepetitive events that could be well-genotyped across the analysed populations. A large fraction of our data set, 3,739 (42%), was deletions of at least a thousand bases in length. This set was also significantly larger (when counting variants larger than 100 bps) than those analysed previously [14] , [15] , [16] , [24] , [25] ( Supplementary Table 1 ). Overall, 4,583 (51%) of deletions intersected 2,706 GENCODE annotated genes, which included 2,498 protein-coding genes and 1,487of their exons. We further classified the deletions by their likely mechanism of origin using sequence signatures at breakpoints from the following classes [14] : NAHR, TEI and non-homologous (NH) events. Note that our set does contain bona fide insertions relative to ancestral state, such as transposable elements [14] . In particular, majority of the TEIs are insertions of Alu elements. The final set consisted of 13% NAHR, 25% TEIs and 61% NH deletions. Large fraction of NH deletions (58%) had evidence of being generated though template-switching mechanisms, that is, contained at least 2 bp identity around breakpoints or MI longer than 10. The remaining NH deletions are likely to arise through NHEJ. Several of the MIs suggested the involvement of transposable elements via non-canonical insertion mechanisms. For example, the MI of one deletion (chr1:200,258,970–200,259,149) consisted of the sequence of 3′-end of an active Alu element and 21-bp-long poly(dA) tail, and is thus likely templated from RNA of an Alu element [26] . We also identified a deletion (chr17:1654955–1655422) generated with a breakpoint signature indicating recombination across the right arm monomers of two oppositely oriented Alus [27] . Overall, the deletions in this set were generated though a variety of mutational mechanisms. We provide this data set as a public resource ( Supplementary Data 1 and http://sv.gersteinlab.org/phase1bkpts ) with complete information about breakpoint coordinates, mechanism classification and, if applicable, the sequence of microinsertions (MIs) at the breakpoint. The resource can be used in various ways including SV genotyping by mapping reads to breakpoint junction sequences. To this end, we extended BreakSeq [14] , [28] , a junction-mapping algorithm for SV detection, into BreakSeq2 for rapid and enhanced SV genotyping ( Supplementary Fig. 4 ). BreakSeq2 supports the SAM/BAM file format and is able to utilize more reads for mapping to sequence junctions. It estimates the zygosity of the calls to provide more information for interpretation. We benchmarked BreakSeq2 breakpoint genotyping on a high-fidelity synthetic genome [29] and on a deep-sequenced human genome of an individual [30] . BreakSeq2 applied (see Methods) with the new, extended breakpoint library is able to genotype roughly ∼ 2,000 SVs per individual with 80–90% sensitivity, double compared with the previous version [14] , while maintaining a high precision of over 98% ( Supplementary Data 2 ). Variant co-aggregation with deletion breakpoints To analyse the association of variants with deletion breakpoints, we aggregated SNPs and indels found in the same group of individuals around breakpoints. To reduce the contamination of our analysis with false-positive calls, we only used variants that reside in confident sites, as defined by the mask of the 1000 Genomes Project [21] , and calculated densities with respect to the number of such sites. Normalized densities (see Methods) of both SNPs and indels increased in the 400-kbp regions around breakpoints of each class ( Fig. 2a and Supplementary Fig. 5 ). One might suggest that false SNP calls as a result of read mis-mapping around breakpoints could cause the observed increase, as reads spanning the SV junctions are often misaligned. However, the increases have a scale that is large relative to the 450- to 650-bp insert size of sequencing libraries and, therefore, cannot be artifactual. Analysis of sequence conservation around breakpoints revealed that these increases could likely be explained by the co-occurrence of different variants in genomic regions under reduced selection. This is evident by the aggregated conservation score decreasing around breakpoints in conjunction with an increase in SNP densities. 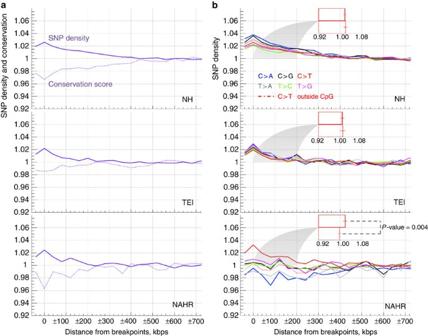Figure 2: Co-aggregation of SNPs with deletion breakpoints found in the analysed samples. (a) Normalized SNP densities increased while conservation decreased in 400-kbp regions around breakpoints of each class. (b) Densities increase for substitutions of all types around NH and TEI breakpoints but this is not the case for NAHR breakpoints. Increase of C to T substitutions around NAHR breakpoints is driven by SNPs in CpG motifs as evident from red bars. Furthermore, this is solely due to enrichment of CpG motifs (Supplementary Fig. 6). This is consistent with common knowledge that NAHR events are associated with sites of recombination. Figure 2: Co-aggregation of SNPs with deletion breakpoints found in the analysed samples. ( a ) Normalized SNP densities increased while conservation decreased in 400-kbp regions around breakpoints of each class. ( b ) Densities increase for substitutions of all types around NH and TEI breakpoints but this is not the case for NAHR breakpoints. Increase of C to T substitutions around NAHR breakpoints is driven by SNPs in CpG motifs as evident from red bars. Furthermore, this is solely due to enrichment of CpG motifs ( Supplementary Fig. 6 ). This is consistent with common knowledge that NAHR events are associated with sites of recombination. Full size image Besides the overall SNP density, the densities of all individual substitution types (for example, C to A) also increase close to NH and TEI breakpoints ( Supplementary Table 2 ). However, this is not the case for NAHR breakpoints, for which C to A and T to A are depleted, while C to T substitutions are enriched ( Fig. 2b and Supplementary Table 2 ). We hypothesized that the observed differences in SNP aggregation can be explained by the sequence and motif content around breakpoints of each class and/or different selection pressure acting on substitutions of each type. Indeed, further analysis, performed by removing CpG dinucleotides from consideration, revealed that the increase in C to T substitutions is due to the enrichment of the CpG motif exclusively around NAHR breakpoints, but not around NH or TEI breakpoints ( Fig. 2b and Supplementary Fig. 6 ). This is expected, as it is known that the motif itself, C to T mutations within it, and NAHR breakpoints are associated with recombination hot-spots [31] , [32] . Indeed, NAHR breakpoints in our set were strongly associated with higher recombination rates (enrichment of 1.4 with P value<10 −3 , Bonferroni Correction), while no significant association for breakpoints of other classes was observed (see Methods). However, unexpectedly, the density of C to T substitutions in CpG motifs decreased close to NAHR breakpoints ( Supplementary Fig. 6 ). Since such substitutions are methylation-associated, we directly tested for DNA methylation levels around breakpoints. Association with epigenome and chromatin states DNA methylation levels from H1ESC line showed no change close to breakpoints of all classes ( Supplementary Fig. 7 ). We next searched for an association of breakpoints with hypomethylated regions in sperm as compared with H1ESC [33] . A strong association was observed for TEI and NAHR breakpoints ( Fig. 3a ). In particular, the TEI breakpoints were five times and NAHR breakpoints were over 50% more likely to reside in hypomethylated regions than expected by chance (both P -values<2 × 10 −4 , see Methods). Such an enrichment for TEI (mostly Alus ) could reflect the long-standing observation of demethylation of Alu elements in sperm [34] . Alternatively, the enrichment could reflect a preference of transposon integration complexes for hypomethylated DNA, as has been observed in somatic TEIs in cancer genomes [35] . Similar enrichment for NAHR deletions is consistent with the reduced C to T substitution densities in CpG regions around the deletions’ breakpoints. This observation is not confounded by CpG islands, most of which are also constitutively unmethylated in sperm ( Supplementary Fig. 8 ). 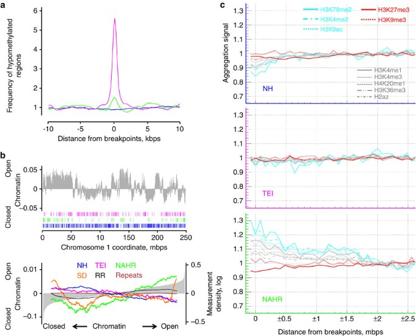Figure 3: Relation of breakpoints of each class to epigenome and chromatin states. (a) Overlap of breakpoints with hypomethylated regions in sperm. NAHR and TEI breakpoints show strong association. (b) Breakpoint co-occurrence with chromatin states, defined by corresponding eigenvector of Hi–C data (upper panel). The genome-wide co-occurrence is ordered by the value of the eigenvector (lower panel). Curves were smoothed using sliding window of 3,000 bins. NAHR breakpoints are associated with open chromatin. This association cannot be explained by higher content of SDs, repeats or recombination rate (RR). (c) Association with histone marks. NH breakpoints were depleted for all active marks and also for the H3K9me3-repressive mark (red lines). TEI breakpoints showed weak depletion of active marks. While the density of repressive H3K27me3 mark decreases close to NAHR breakpoints, the density of all active marks increases. Figure 3: Relation of breakpoints of each class to epigenome and chromatin states. ( a ) Overlap of breakpoints with hypomethylated regions in sperm. NAHR and TEI breakpoints show strong association. ( b ) Breakpoint co-occurrence with chromatin states, defined by corresponding eigenvector of Hi–C data (upper panel). The genome-wide co-occurrence is ordered by the value of the eigenvector (lower panel). Curves were smoothed using sliding window of 3,000 bins. NAHR breakpoints are associated with open chromatin. This association cannot be explained by higher content of SDs, repeats or recombination rate (RR). ( c ) Association with histone marks. NH breakpoints were depleted for all active marks and also for the H3K9me3-repressive mark (red lines). TEI breakpoints showed weak depletion of active marks. While the density of repressive H3K27me3 mark decreases close to NAHR breakpoints, the density of all active marks increases. Full size image Next, we used two states of the chromatin interactome, as defined by Hi–C experiments [36] , roughly corresponding to open and closed chromatin, to investigate any correlation of breakpoints with open and active DNA chromatin. We tested for the occurrence of breakpoints in genomic bins of 100 kbps assigned to either state. To determine the significance of our findings we fixed relative arrangements of chromatin states and the relative arrangement breakpoints, but randomized positions of the states and breakpoints with respect to each other (see Methods). We observed ( Fig. 3b ) that NH and TEI breakpoints are depleted for open chromatin, while NAHR breakpoints are enriched ( P -value<10 −4 , Bonferroni Correction). Segmental duplications (SDs) are known to mediate NAHR. We indeed ( Fig. 3b ) saw a positive correlation (Spearman coefficient, 0.85) between NAHR and SDs but only in the closed chromatin, while in the open chromatin we observed a negative correlation (Spearman coefficient, −0.32). Similarly, we observed a strong correlation of recombination rate with NAHR breakpoints in closed chromatin (Spearman coefficient, 0.94), but significantly weaker correlation in the open chromatin (Spearman coefficient, 0.28). This suggests two conditions for generating deletions by NAHR. We further analysed an association of breakpoints with 10 chromatin marks ( Fig. 3c ). The three classes of breakpoints showed very different associations. NH breakpoints were depleted for all active marks and also for the H3K9me3-repressive mark. TEI breakpoints showed weak depletion of active marks. However, NAHR breakpoints were characterized differently. The density of repressive H3K27me3 mark decreases close to NAHR breakpoints, while the densities of all active marks increase. As active marks are linked to open chromatin [36] , these observations corroborate the association of NAHR with open chromatin. Hi–C data and chromatin marks define open chromatin on a large kilobase to megabase scale, while accessible DNA, which is a subset of open chromatin, can be defined on the scale of a few hundred and dozen bases. We correlated our breakpoints with DNase-hypersensitive sites and with nucleosome-free DNA ( Supplementary Fig. 9 ). DNase data revealed association of NAHR breakpoints with accessible DNA at a kilobase range. Nucleosome occupancy data further uncovered preference of NAHR breakpoints to reside in nucleosome-free regions. Analysis of the both data types revealed no association with NH breakpoints, but depletion of TEI breakpoints in nucleosome occupied and DNase-accessible regions. Breakpoint deletions and their relation to replication timing Multiple studies have reported the existence of microinserted sequences at deletion breakpoints. In our data set we observed 2,391 (27%) deletions with MI ranging in length from 1 to 96 bps, with the majority being less than 10 bps in length ( Fig. 4a ). Those could arise from technical ambiguities in breakpoint reporting when there are SNPs or indels close to breakpoints (see Methods). We therefore focused the following analyses on MI longer than 10 bps. 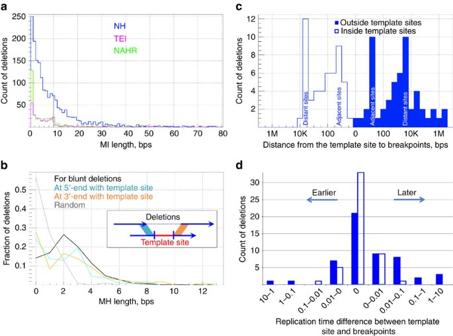Figure 4: Analysis of MI at deletion junctions. (a) MI up to 10 bps in length could arise from technical ambiguities in breakpoint reporting when there are SNPs or indels close to breakpoints. Larger MIs are typically found for NH deletions. (b) Length of microhomology (MH) at deletion junction. For deletions with MIs and identified template site, MHs are calculated for 5′-ends/3′-ends of the deletion and the template site (panel insert). Both ends show MI longer than expected by chance and similar to the distribution for blunt deletions. (c) The distribution of the nearest distance from template site breakpoints in the log10scale. The distribution is almost symmetrical and exhibits distinct peaks between 20 and 60 bps (adjacent sites) and between 2 and 6 kbps (distant sites). (d) The difference in replication time between the template site and breakpoints reveals later replication of template sites. For template sites outside the deletion the effect is significant (P-value<0.03 by binomial test). The effect is even more significant (P-value<0.01) when excluding difference of up to 0.01, as such small values are comparable to measurement error. Figure 4: Analysis of MI at deletion junctions. ( a ) MI up to 10 bps in length could arise from technical ambiguities in breakpoint reporting when there are SNPs or indels close to breakpoints. Larger MIs are typically found for NH deletions. ( b ) Length of microhomology (MH) at deletion junction. For deletions with MIs and identified template site, MHs are calculated for 5′-ends/3′-ends of the deletion and the template site (panel insert). Both ends show MI longer than expected by chance and similar to the distribution for blunt deletions. ( c ) The distribution of the nearest distance from template site breakpoints in the log 10 scale. The distribution is almost symmetrical and exhibits distinct peaks between 20 and 60 bps (adjacent sites) and between 2 and 6 kbps (distant sites). ( d ) The difference in replication time between the template site and breakpoints reveals later replication of template sites. For template sites outside the deletion the effect is significant ( P -value<0.03 by binomial test). The effect is even more significant ( P -value<0.01) when excluding difference of up to 0.01, as such small values are comparable to measurement error. Full size image As in previous studies [15] , [16] , MIs were observed almost exclusively (83%) for NH events. It has been suggested that template-switching mechanisms during replication generate deletions with MI that are copies of some sequence in the genome [13] . To test for this possibility we determined the likely genomic origin, that is, the template site, of 133 inserted sequences of which 114 were 20 bps or longer, constituting 42% of all MIs of such length ( Supplementary Data 3 ). Other MIs did not map to the reference genome, mapped only partially or mapped to multiple locations. We categorized template sites as those (i) within a deletion, which were 49 (37%) in total; (ii) outside of a deletion, but on the same chromosome, totalling 52 (39%); and (iii) on a different chromosome, totalling 25 (19%). Seven template sites spanned breakpoints and were excluded from analysis. It was previously observed that NH events typically have few bases of homology around their breakpoints and template sites [14] , [15] , [16] , [37] . We do confirm this observation ( Fig. 4b ) for blunt deletions and those 101 template sites located on the same chromosome as the corresponding deletion. However, no sequence microhomology around breakpoints was apparent for deletions having template sites on different chromosomes ( Supplementary Fig. 10a ). The distribution of the nearest distance between the template site and either of the breakpoints revealed preferred relative arrangement ( Fig. 4c ). The template site was typically located either between 20 and 60 bps (adjacent site) or between 2 and 6 kbps (distant site) of one of the breakpoints. The existence of such characteristic distances may signify the mechanism(s) leading to the generation of MI. It was previously noted [38] that breakpoints of deletions generated by different mechanisms are associated with different replication times. We confirm those observations: NAHR deletions are typically associated with early replicating regions, NH with later ones, while TEIs show no significant relation to replication time. Furthermore, template sites outside deletions typically replicate later ( Fig. 4d ) than breakpoint regions ( P value<0.03 by binomial test). However, the same effect was not significant for template sites within deletions, possibly due to low resolution of the replication time measurement, which is of kbp scale. Similarly, we did not see preference for later or earlier replication times for template sites on different chromosomes ( Supplementary Fig. 10b ). In this study we derived a large set of germline deletion breakpoints. This set represents deletions across a broad length scale, with high quality of breakpoint sequences, and across three likely mechanisms of origin, thereby allowing us to categorize breakpoints into three classes: NH, NAHR and TEI. It should be noted that NAHR and TEI events are more difficult to discover as they contain repeats, and so are likely to be under-represented in this set. Further analysis revealed that a common feature for breakpoints of all classes is the association with evolutionarily less conserved genomic regions, spanning up to hundreds of kilobases downstream and upstream of the breakpoints. This is likely due to purifying selection disfavouring deletions. Selection is likely the reason explaining co-occurrence of breakpoints in each class with SNPs. Alternatively, one can suggest that genomic features (for example, nucleosome-free DNA) that predispose to certain classes of SNPs may also predispose to certain classes of SVs. While indeed we see such associations (for example, for NAHR breakpoints), except for reduced conservation, we did not find any other feature that would be universally associated with breakpoints in each class. Associations with other measures—CpG motif density, various types of nucleotide substitutions, histone marks, open chromatin, accessible DNA, methylation and replication time—were different between deletion mutation mechanisms. The classical NAHR mechanism postulates meiotic cell division as a requirement for generating a germline SV. This implies certain associations that we did observe in our study. In particular, NAHR breakpoints were associated with higher recombination rates, with higher GC content and with higher density of CpG motifs. However, and unlike other classes, they were also associated with open chromatin, higher DNA accessibility and active histone marks in mitotically dividing cells. This poses a paradox. No defined structure of DNA exists at the time of chromosome segregation [39] and histone marks are gone [40] ; thus, no association of breakpoints with open/active chromatin is expected. In fact, as a result of purifying selection one might expect an inverse relation of breakpoints with open chromatin and active histone marks, such as in the case of NH breakpoints. Neither recombination rate nor the fraction of bases in SDs or in repeats explain these associations for NAHR breakpoints. The association of NAHR with early replication timing is also stunning. By the time of chromosome segregation, DNA replication is complete and replication time should not play a role. In addition, we found two lines of evidence associating NAHR breakpoints with hypomethylation: lower frequency of C to T SNPs in CpG motifs and an enrichment with demethylated regions in sperm. NAHR breakpoints have been previously suggested to be associated with hypomethylation [41] ; however, the findings were debated with the notion that technical variability may explain the association [42] . In our SNP aggregation analysis, we used roughly 70% of the human genome sequence where SNPs could be confidently determined. Demethylated regions in sperm used in our study were determined from comparative analysis of methylation profiles that are directly inferred from whole-genome bisulfide sequencing in sperm and embryonic cell. Such comparative analysis is not likely to be influenced by technical artefacts. We, thus, state that the observed association of NAHR breakpoints with hypomethylation is not artefactual, although not as strong as suggested in ref. 41 . It also corroborates association of NAHR breakpoints with open chromatin. On the basis of all these observations, we hypothesize that a fraction of SVs mediated by NAHR could originate in germ cells and early embryonic cells without replicating DNA and dividing. Open/active chromatin contains unpacked DNA that is easy to melt and may contain single-stranded DNA, for example, as a result of transcriptional activity. Such DNA can serve as a template in double-stranded break repair pathway for breaks in homologous region(s) that are close in space and thereby likely to be from the same chromosome [36] . In fact, intramolecular NAHR, which is homologous recombination between regions of the same continuous chromosome, has been previously suggested [43] , [44] , and the consequence of such an event would be generation of a deletion and a piece of extrachromosomal circular DNA (eccDNA). eccDNA was recently extensively analysed [45] in mouse somatic tissues and human cancer cell lines. The striking observation was that eccDNA was enriched in CpGs and exons, supporting the suggestion that unpacked DNA is a requirement for eccDNA generation. The length of eccDNA circles was typically 200–400 bps, but could be as long as 2,000 bps, consistent with a median of 418 bp for NAHR deletions in our set. The association with early replication timing in our hypothesis is transient through open chromatin, which replicates first [46] . The association of TEI breakpoints with SNP density, conservation, open chromatin and histone marks was similar to that of NH breakpoints, but less pronounced. We think this is due to TEIs, as bona fide insertions are likely to disrupt only a few bases around insertion sites and, thus, are less likely to have deleterious effect as compared with NH deletions spanning from hundreds to millions of bases. TEI association with hypomethylation in sperm could be due to a known phenomenon [34] or could imply preference for insertion into hypomethylated DNA [35] . Distinguishing these possibilities will require further study. Besides possible association of methylation with TEIs, we observed strong correlation of transposable elements with nucleosome-free DNA. This observation is consistent with the notion that nucleosomes are generally refractory to nicking by human L1 reverse transcriptase, the key enzyme for retrotransposition [47] . Our analysis also provided insight into the mechanism(s) of generating deletions in the NH class. Such deletions are thought to originate from NHEJ and template-switching mechanisms during replication, such as fork stalling and template switching or microhomology-mediated break-induced replication. The template-switching mechanisms predict [13] that a replication fork can accidentally switch sites of template DNA during DNA duplication. Switching sites skip some genome sequences, thereby generating deletions, or re-replicate the same sequence, thereby generating duplications. MIs are generated at breakpoints when switching occurs more than once. We found that template sites for MIs have sequence microhomology at breakpoints, are located at two characteristic distances from breakpoints (between 20 and 60 bps—adjacent and between 2 and 6 kbps—distant) and replicate later than the regions of breakpoints. In about half of the cases, template sites were within breakpoints of corresponding deletions. One might explain such cases by the co-occurrence of two deletions (or of a deletion and an indel), generated in different individuals (possibly by different mechanisms) and eventually integrated on the same allele and discovered as a single deletion. In other words, it might be suggested that MIs are genomic sequences between two adjacent variants. We think that such an explanation does not apply to most cases. The distributions of the nearest distance to breakpoints for sites within and outside breakpoints are very similar and both have the same two characteristic distances. This suggests that deletions with MI template sites within and outside breakpoints are generated by the same mechanism, for example, by template switching. As template sites from outside deletions could not be explained by variant co-occurrence, we argue that template sites within deletions could not be explained by variant co-occurrence either. We also observed that template sites at different chromosomes do not have sequence microhomology at breakpoints and are not replicating later or earlier as compared with breakpoints. This may imply that MIs with template sites on the same and different chromosomes are created by different mechanisms; for example, MI was copied from RNA transcribed from distant region [26] , as we found one such event. It is also possible that template sites on different chromosomes arise from mis-mapping the sequences of MI. We further hypothesize that the distance to template sites could be related to DNA packing in a cell during replication. For example, larger characteristic distances could reflect the length of DNA when wrapped with one loop around the replication bubble to bring a template site close to a collapsed or stalled replication fork. The later replication times of template sites suggest that it would still be in the form of a double helix and when dissociated, perhaps by another replication bubble, could provide the template sequence for template switching by the collapsed or stalled fork. Large high-quality breakpoint data set significantly empowered our analysis. For example, 133 mapped template sites of MIs constitute only 1.5% of all breakpoints in our set. Previous studies dealt with smaller sets, and a similar analysis was not feasible. Future studies will have larger and more comprehensive, including for duplications and inversions, breakpoint sets. Thus, it is likely that our knowledge of mutational mechanisms for SVs will be further expanded and refined. Deletion discovery and merging and breakpoint inference Deletions discovered by five copy number variation (CNV) callers [48] , [49] , [50] , [51] , [52] were merged with the set of breakpoints discovered in 180 pilot samples of the 1000 Genomes Project [17] . The merged set contained 113,649 deletion calls. For each call we collected read pairs around its boundaries in samples where the deletion was discovered and assembled them with TIGRA-SV [22] into contigs spanning breakpoints. The contigs were aligned to the deleted regions with CROSSMATCH and AGE [23] to identify deletion breakpoints (see below). This way we inferred 36,237 breakpoints, of which 17,947 (50%) breakpoints were exactly the same by the two approaches, 9,537 (26%) breakpoints were different by the two approaches and 8,753 (24%) were uniquely inferred by either one of the approaches. In cases where the two approaches inferred different breakpoints, we chose breakpoints from AGE alignments, as the AGE method was specifically designed to align contigs with SVs. Because of disagreement between the two approaches, we further filtered breakpoints by aligning unmapped reads to sequence junctions of the deletions (see below and Fig. 1 ). On the basis of PCR validation, we performed an additional filtering of deletions to reduce systematic false-positives arising from the use of synonymous split-read (SR) approaches: deletion calling by SR, breakpoint derivation from assembly (which is SR-based) and filtering from read mapping to junction (which is SR-like). To summarize, all filtering steps were as follows: (i) removing breakpoints not passing criteria for support by mapped reads to their junction (see below); (ii) removing deletions classified as variable number of tandem repeat, as their breakpoints are in very repetitive regions; (iii) removing breakpoints only found by SR calling approaches Delly, Pindel and assembled in the pilot (the reason being that in the case of a mistake by a discovery method, assembly/filtering could repeat it, because it relies on a SR approach); (iv) removing deletions with breakpoints inferred from only CROSSMATCH alignments; (v) removing deletions called by only one method with breakpoints inferred from only AGE alignments. The first three filters were the most effective in removing false-positive calls ( Supplementary Fig. 11 ). The final set consisted of 8,943 deletion breakpoints with consistent FDR estimates from PCR (6.8%) and IRS (6.4%) tests for deletion presence, and 13.7% for deletion with correct breakpoints from PCR. FDR for deletion breakpoints includes mistakes when deletion is not present, but also includes cases in which the breakpoint is incorrectly determined ( Supplementary Fig. 1 ). Around 16% of deletions were present in only one initial call sets merged ( Supplementary Fig. 11 ), stressing that the majority of deletion sites were detected by multiple algorithms. Defining breakpoints from CROSSMATCH alignments For a contig assembled from an intrachromosomal variant in the genomic interval [ a,b ], we prepared a local reference sequence excised from [ a − w , b + w ], with w =500 bp by default. For a contig assembled from an interchromosomal rearrangement, we prepared two local reference sequences from [ a − w , a + w ] of chromosome c1 and from [ b − w , b + w ] of chromosome c2, respectively. We mapped each contig assembled by TIGRA to the corresponding reference sequences using CROSSMATCH. In the default setting, we used the following CROSSMATCH parameters: -bandwidth 20 -minmatch 20 -minscore 25 -penalty -10 -discrep_lists -tags -gap_init -10 -gap_ext -1. We removed contigs that had more than two hits to the reference and ignored alignments that had substitution rates greater than 0.5%. If a contig differs substantially from the reference, CROSSMATCH returns multiple local alignments, together with a set of statistics describing the quality of the alignments. A glocal alignment (combination of local and global alignment) was constructed from these local alignments [53] . We used that alignment as the basis for reporting the existence of breakpoints and details about the type, size, orientation and location of the breakpoints ( Supplementary Fig. 12 ). For example, the glocal alignment that supports a deletion breakpoint contains two local 1-monotonic alignments to the reference [54] . The gap between the end position of the first alignment and the start position of the second alignment corresponds to the size of the deletion, while the bases shared by both alignments correspond to breakpoint homology. Defining breakpoints from AGE alignments Contigs assembled by TIGRA-SV at least 100 bps in length were aligned to the corresponding predicted deleted region extended by 2 kbps downstream and upstream. AGE was run with options ‘-indel –match=1 –mismatch =−10 –go=−10 –ge=−1’, which specifies that contigs or reference regions are expected to have large insertions/deletions; that the score for base match is 1; that the mismatch penalty is −10; that the gap opening penalty is −10; and that the gap extension penalty is −1. Alignments consistent with the predicted deletion were selected to identify deletion breakpoints. The consistency was defined by the following criteria: (i) at least 90% of bases in a contig are aligned; (ii) there must be at least 98% of identical bases in an entire alignment; (iii) there should be at least 97% identical bases in alignment of each flank, that is, downstream or upstream from the deletion; (iv) each flank must have at least 30 base pairs aligned; (v) regions between breakpoints must have 50% reciprocal length overlap with the predicted deletion bounds; (vi) breakpoints should be within 200 bps of the predicted deletion bounds; (vii) alternative alignments, if any, must satisfy all of the conditions above. In case of multiple contig alignments satisfying the above conditions, the one with the contig of highest coverage, as per assembly, was chosen to define breakpoints. Filtering breakpoints by mapping to breakpoint junctions Most of the reads utilized in assembly were from 30 to 70 bps in length, that is, rather short. This fact complicates assembly and makes it rather prone to mistakes, particularly in repetitive regions, for which deletion breakpoints are enriched. Therefore, to ensure physical (rather than artificial, as a result of assembly error) continuity of flanking and inserted (if any) sequences at breakpoints, we performed breakpoint filtering by utilizing unmapped reads. For each derived deletion breakpoint we constructed a breakpoint junction sequence by joining 100 bps downstream with 100 bps upstream of the breakpoints. The MI (if present) was inserted in the middle. The set of all 36,237 junctions sequences from 200 to 298 bps in length comprised the junction library. Unmapped reads were mapped to the junction library using Bowtie 0.12.7 (ref. 55 ) with the options ‘--best --strata -v 3 -m 1’, requiring that ungapped alignments are made with at most three mismatches and that only unique alignments are reported. Before mapping, and in the same way that it was performed by BWA [56] during alignment preparation by the 1000 Genomes Project, the reads were trimmed at low quality 3′-end up to the average base quality of 15. Reads mapping with less than 3% of mismatches of their length and having aligned bases in downstream and upstream flanking sequences were considered in potential support of the junction they aligned to. We chose a particular cutoff d on the number/fraction of bases aligned to each flank for deciding, which reads supported breakpoints. Breakpoints that had supporting reads from two different individuals passed the filter. This requirement ensures that breakpoints passing the filter are for heritable germline deletions, as singletons could be of somatic origin. In total, we attempted realigning 15.8 billion reads to the junction library. Given the large number of realigned reads and the large size of the junction library, some of the read mappings could have been mapped by chance. To discriminate between real and random mappings we developed an empirical null model ( Fig. 1b ). The model is based on imitating the junction library with semi-random sequences, thereby creating a null junction library, and mapping unaligned reads to that null library. Such a mapping will represent random noise and can be used for optimizing values of d . The library is generated from inner sequences of deleted regions ( Fig. 1b ). Such an approach is advantageous in that it allows preserving genomic (for example, nucleotide content and sequence homology at breakpoints) and data features (for example, read coverage) associated with the loci of breakpoints. We realigned all unmapped reads to the null junction library and varied the values of d to find the cutoff at which the number of null junctions passing the filter was <5% of the number of real junctions passing the filter at the same cutoff ( Supplementary Fig. 13 ), that is, we aimed for <5% in silico FDR. This criterion led to setting the value of d at 13 bps. The empirical null model allowed us to stratify the precision of breakpoint by various categories. For example, and as expected, we observed that breakpoints found by only one approach (either AGE- or CROSSMATCH-based) have higher in silico FDR. The order of breakpoints of different classes by corresponding in silico FDR was (from lowest to highest): NH, TEI, NAHR and VNTR. This is also expected, as breakpoints of different classes have progressively more repeats around their breakpoints in the same order. To summarize, we developed an empirical model that captures essential biological features of breakpoints, that is not biased because it uses data loci different from the breakpoints, and that allows the translation of random mappings into an estimated FDR. We suggest that such empirical models can be used to estimate FDR of genotyping known breakpoints from sequencing data. However, when it is applied to breakpoint filtering/validation, one should keep in mind that the approach may not account for systematic false-positives arising during structural variant calling by SR method(s), as was observed in our analysis (see above). PCR and IRS validations We selected 15–22 deletions of each class for PCR validation. Deletions were selected randomly, but required to be genotyped in at least two samples out of 319 for which we had DNA available. Here we relied on genotyping by mapping reads to deletion breakpoint sequence junctions. For the selected deletions we designed primers with Primer3 such that the primers would amplify the breakpoint sequence. For each deletion we ran PCR in at least one sample genotyped as having it and sequenced the resulting band with Sanger technique. In case the deletion was not confirmed, we ran the PCR in another sample genotyped as having it (the deletion). IRS validation [17] was as follows. Briefly, the validation considers intensities of SNP probes within deleted regions and correlates it with deletion genotypes across samples. It is expected that for such SNPs, samples with deletion will have lower intensity values than samples without the deletion. Rank sum tests are performed to access the statistical significance of correlations. IRS only tests the validity of deletion sites and does not provide validation of breakpoints. Results of performing these exercises are summarized in ( Supplementary Fig. 11 ). Comparing with OMNI genotypes A set of 11,472 breakpoints derived in the pilot of the 1000 Genomes Project was tested on a custom SNP array designed by ILLUMINA and named OMNI 2.5 s array. The pairs of probes were designed such that one probe would hybridize to the reference allele and the other one to the breakpoint sequence, that is, to the alternative allele. The probes were different in only one nucleotide to mimic probes for SNP genotyping. Accordingly, all the downstream hybridization signal processing was performed with standard software for SNP array analysis. Probe design, hybridization in 431 individuals and genotyping quality control resulted in confident array-derived genotypes for 4,385 (38%) breakpoints. Overall, 2,483 of our confident breakpoints were in this set ( Supplementary Data 1 ) and 292 individuals were both sequenced by the 1000 Genomes Project and genotyped by this array. Comparison of samples genotyped (by the array) as having a deletion to those carried out by mapping reads to sequence junctions, as we did for filtering breakpoints, revealed that individuals with deletion genotypes by read mapping represent almost a perfect subset of those genotyped by arrays ( Supplementary Fig. 2 ). This is easy to rationalize by noting that individuals in the 1000 Genomes Project were sequenced at a shallow 4–8X coverage, and thus not likely to have many reads covering breakpoint sequences, particularly in the case of heterozygous deletions. Furthermore, the requirement that reads mapped to deletion sequence junction must extend at least 13 bps across the junction in each direction, further reduces the number of reads that we consider supporting deletions. Confirmation of breakpoints in high coverage trios Breakpoint confirmation was performed using data for two trios sequenced with HiSeq 2500 at 60 × coverage with 250-bp reads. The 8,943 deletions in our confident set were genotyped in trios by CNVnator [48] , and when genotypes suggested the presence of deletions (estimated copy number less than 1.5 or less 0.5, for diploid and haploid regions, respectively), corresponding breakpoints were selected for further investigation. Read pairs with coordinates in the 2-kbp vicinity of these regions were extracted from BAM files, and each pair was tested for an overlap at 3′-ends. If a suitable overlap was detected, the reads were merged into a long continuous (gapless) genomic fragment. The reads in the HiSeq 2500 data were 250 bp in length, with an average insert size of ∼ 400 bp ( Supplementary Fig. 14 ). This means that the reads in most read pairs significantly (50 bp or more) overlapped in sequence at the 3′-ends. In our validation method, we merged overlapping read pairs to construct long genomic fragments. To merge a given pair aligned near deletion breakpoints, we needed to estimate the length of its overlapping sequence. We slid the 3′-ends of each read in a pair against each other starting from an overlap of 1 base and continuing up to 250 bases. For a given overlap of length n , we assumed a binomial distribution for the number of mismatches. We selected overlap lengths that minimized the P -value under this assumption, that is, given k mismatches in a overlap of length n , the probability that at most k mismatches would occur by chance with the uniform probability for each mismatch of P mismatch =0.75. We only considered merged read pairs that had mismatch counts less than 20% of overlap length, and P -values smaller than 10 −10 . We tested our approach by independently aligning overlapping reads and comparing these overlaps to those from alignment. Consistent overlaps were observed for 99.95% of read pairs ( Supplementary Fig. 15 ). Pairs of reads with identified overlaps were merged into genomic fragments, and bases in overlapping sequences were chosen by taking the base with the higher quality score at positions of mismatches. These genomic fragments were from 250 to 480 bps in length and of higher sequencing quality than either of the reads in the original pair alone. Using AGE [23] , we generated split-fragment alignments of such fragments around breakpoints and searched for breakpoint support the same way we did for contig alignment with AGE (see above). We considered breakpoints with such supporting reads as at least partially confirmed. We considered a given breakpoint to have perfect support if read alignments had breakpoint coordinates and microinserted sequences (if any) that matched exactly. A breakpoint was considered confirmed if the majority of split-fragment alignments, consistent with the deletion, matched the breakpoints perfectly. We confirmed 3,034 (34%) breakpoint sequences perfectly and, for 423 (4.7%) more, we observed slight differences in the sequence at breakpoints. Our ability to confirm breakpoints was confounded by incorrect genotypes (that is, deletion not present in a sample but genotyped as such), as we observed a lower confirmation rate for smaller deletions ( Supplementary Fig. 16 ). An additional confounding factor was the limited ability to construct long reads, because the 3′-ends had high sequencing error, and reliable overlap for paired reads could not be found. In particular, less than 30% of considered pairs of reads have an identifiable overlap. Therefore, unconfirmed breakpoints could be categorized as: (i) just false breakpoints; (ii) true breakpoints but with incorrect genotype; or (iii) true breakpoints with correct genotype, but with no constructed long reads covering the junction. To estimate FDR of the set we minimized the number of breakpoints in the latter two categories by considering deletions larger than 10 kbp and genotyped in at least three individuals. This resulted in a FDR estimate of 18% for deletion presence with correct breakpoints. Aggregation calculation Almost 40 million of SNPs and indels found by the 1000 Genomes Project [21] in the same group of individuals were aggregated around the breakpoints of each class. To reduce the contamination of our analysis with false-positive calls, we only used SNPs and indels that reside in the confident sites as defined by the mask derived by the project. This reduced the number of variants by 25%. SNP density was calculated with respect to the number of such sites. Densities of substitutions at C and G bases were calculated with respect to the number of not masked C and G sites. Densities of substitutions at A and T bases were calculated with respect to the number of not masked A and T sites. Each aggregated density was then normalized to yield density of one in the interval (±500 kbps, ±1 Mbps). Histone mark data generated by the ENCODE [19] project were used for the aggregation analysis. We utilized contained normalized histone signals provided by the project. Aggregated signal in each bin was normalized with respect to number of available bases, that is, undetermined bases of the reference genome were excluded from the aggregation. Each aggregated signal was then normalized to have value of one in the interval (±2 Mbps, ±4 Mbps). We utilized methylation data generated with bisulfide sequencing by The NIH Roadmap Epigenomics Mapping Consortium [20] . The data were provided for only those CpG sites where confident methylation level estimation could be made, which is ∼ 95% of all CpG sites. Aggregated methylation levels were then normalized to the number of CpG sites. Intersection with open or closed chromatin We used the Hi–C data generated on the human lymphoblastoid cell line (GM06990) (ref. 36 ). In that study, chromatin states were defined from chromatin interaction matrix eigenvectors that correspond to chromatin states. The matrix was calculated for consecutive nonoverlapping genomic bins of 100 kbs in length: negative values represent closed chromatin states, and positive ones represent open states. There were a total of 28,481 bins with non-zero eigenvector values. We assigned each breakpoint with an eigenvector value by finding the bins they belong to. NAHR breakpoints have higher eigenvector values, indicating a more open chromatin state. Meanwhile, NH and TEI breakpoints show lower values ( Fig. 3b ). To test this hypothesis, we utilized a nonparametric rank sum test with restricted permutation. Rank sum was defined by the summation of ranks of the eigenvalues of certain breakpoint subtypes. Then the observed rank sum was compared with an empirical distribution generated by a circular permutation. That is, we joined the end of the whole-genome bin array with the beginning to make it circular, and rotated this circular array to every possible position. We calculated the rank sum for each position. This forms an empirical distribution for the null hypothesis. The P -values are corrected by the Bonferroni method for multiple testing, that is, testing for three sets of breakpoints: NH, TEI and NAHR. Nucleosome occupancy and DNase accessibility signals We used the combined DNase peak call set for human embryonic stem cell (hESC) line with 0.01 FDR from the ENCODE project. Then for each 100-bp bin within the 2.5-kb upstream and downstream regions of the breakpoints, we calculated the average number of overlapping base pairs with DNaseI-hypersensitive peaks. The results were reported in the unit of (overlapping) bp per kb region. We used the nucleosome density signal map generated by Mnase-seq from ENCODE/Stanford/BYU on GM12878 cell lines. Then signal in each 10 bp bin within the 1-kb upstream and downstream regions of the breakpoints was aggregated. To normalize the plot, we divided the signal for each bin by the average signal for each breakpoint type. Mapping template sites The majority of MIs are less than 10 bps in length ( Fig. 4a ). Some of these could be explained by the existence of base mismatches or indels close to deletion breakpoints in the aligned contig. Mismatches and indels are penalized and including them in the alignment decreases the overall alignment score, while aligning few bases between the mismatch/indel and breakpoints cannot compensate for the alignment score decrease. As such, an aligner chooses not to align those few bases and reports them as a MI. Given our alignment parameters (see Methods), it is possible that MIs shorter than 10 bps arise because of such an effect. An enrichment of point mutations close to deletion breakpoints has been previously described [37] and was also observed in this study on a larger scale ( Fig. 1 ). We therefore performed the following analyses for MI longer than 10 bps. We first uniquely mapped MIs with up to one mismatch to the reference genome using Bowtie [55] with the following options ‘-n 0 -l 5 -r --best --strata -v 0 -m 1’. Next, not mapped MIs of at least 20 bases in length were aligned to the reference genome by Blat [57] . We then manually examined alignments and selected only one, such that (i) MI is aligned almost full length with few mismatches and/or short indels; (ii) the alignment has much better alignment score than other alignments. In total, we mapped 133 template sites, of which 66 were mapped manually ( Supplementary Data 3 ). Replication time analysis We utilized data by Koren et al. [38] , which had average replication timing from three experiments. Using the data we identified replication time to each breakpoint and template site. Difference in replication time can be calculated relative to each breakpoint. We use the difference that is smaller in absolute value. Calculating association with recombination rates Recombination rate data were derived from the Rutgers third-generation genetic map. We used the sex-averaged genetic positions, ignoring the X and Y chromosomes. Genetic positions were divided by the difference in adjacent physical positions in the map in order to obtain values in terms of centimorgans per basepair (cM per Bp). Linear interpolation was performed to obtain recombination rate values for each base of each chromosome. Significance values were obtained by conducting a circular permutation experiment in the same manner as for intersection with open/closed chromatin (see above). NAHR breakpoints in our set were strongly associated with higher recombination rates (enrichment of 1.4 with P -value<10 −3 Bonferroni Correction), while no significant association for breakpoints of other classes was observed ( Supplementary Fig. 17 ). BreakSeq2 The original BreakSeq approach demonstrated the proof of principle that SVs can be identified from mapping short reads to their breakpoint sequence junctions. In the BreakSeq2 we elaborated on this principle and developed functionality for breakpoint genotyping. Substantial enhancements ( Supplementary Fig. 4 ) of BreakSeq2 are as follows (i) utilization of a larger library, as compared with the original one ( Supplementary Data 2 ); (ii) utilization of more reads for mapping to breakpoint sequence junction ( Supplementary Fig. 4 ); (iii) leveraging the information content captured in the alignment to sequence junctions ( Supplementary Fig. 4 ); (iv) providing SV zygosity estimate. A new and larger breakpoint library utilized by BreakSeq2 was built by combining breakpoints analysed here with extra nonredundant breakpoints from the pilot phase of the 1000 Genomes Project and from the original BreakSeq library ( Supplementary Data 2 ). Breakpoints were considered as redundant if their SV events overlapped 50% reciprocally. We benchmarked BreakSeq2 for its performance on deletion detection. On the basis of a high-fidelity synthetic genome [29] , BreakSeq2, along with the new breakpoint library, increased the sensitivity by almost 15-folds to 85.14% (while maintaining a 98.17% precision), when compared with using the original breakpoint library (<2,000 SVs) with the original BreakSeq ( Supplementary Data 2 ). With a deep-sequenced human genome of an individual [30] , BreakSeq2 attained an average sensitivity of 86.32%, when compared with a three-way consensus call set detected by three other orthogonal SV detection methods ( Supplementary Data 2 ). This is consistent with what we observed in simulation. Overall, BreakSeq2 is highly accurate with the ability to rapidly detect SVs with predicted genotypes. BreakSeq2 is open source and available at http://bioinform.github.io/breakseq2 . How to cite this article : Abyzov, A. et al. Analysis of deletion breakpoints from 1,092 humans reveals details of mutation mechanisms. Nat. Commun. 6:7256 doi: 10.1038/ncomms8256 (2015).